Prolonged spontaneous emission and dephasing of localized excitons in air-bridged carbon nanotubes The bright exciton emission of carbon nanotubes is appealing for optoelectronic devices and fundamental studies of light-matter interaction in one-dimensional nanostructures. However, to date, the photophysics of excitons in carbon nanotubes is largely affected by extrinsic effects. Here we perform time-resolved photoluminescence measurements over 14 orders of magnitude for ultra-clean carbon nanotubes bridging an air gap over pillar posts. Our measurements demonstrate a new regime of intrinsic exciton photophysics with prolonged spontaneous emission times up to T 1 =18 ns, about two orders of magnitude better than prior measurements and in agreement with values hypothesized by theorists about a decade ago. Furthermore, we establish for the first time exciton decoherence times of individual nanotubes in the time domain and find fourfold prolonged values up to T 2 =2.1 ps compared with ensemble measurements. These first observations motivate new discussions about the magnitude of the intrinsic dephasing mechanism while the prolonged exciton dynamics is promising for applications. The photophysics of excitons in single-walled carbon nanotubes (SWCNTs) has been the subject of much recent interest [1] . An appealing property for optoelectronic device applications, as well as fundamental studies, is the weakly screened Coulomb interaction giving rise to exciton-binding energies up to 400 meV (ref. 2 ), which are about an order of magnitude larger than for excitons in II–VI or III–V semiconductor quantum dots. Unlike quantum dots, the photoluminescence (PL) quantum yield in one-dimensional SWCNTs is rather low [3] . It is, however, increasingly understood that this is caused by extrinsic non-radiative recombination of highly mobile excitons exploring defects and dopants along the tube [4] , [5] , [6] , [7] , [8] , [9] , [10] , [11] , and to a lesser extend due to intrinsic exciton dark states affecting PL yields only below 50 K (ref. 12 ). Magneto-optical studies of individual SWCNTs at 20 K reveal directly the zero-field splitting energy Δ x between dark and bright state excitons, which can be well explained by a model of free excitons [13] , while the large scatter of Δ x in tubes of the same chirality was attributed to local variations in the dielectric screening [14] . There is also increasing evidence that excitons can localize randomly along the tube and form quantum-dot-like states [15] , as is indicative from near-field scanning experiments [16] and the observation of photon antibunching at low temperatures [17] , [18] . As a result of these extrinsic effects, dynamical properties of excitons are affected over many timescales in experiments giving rise to PL blinking and spectral diffusion (SD) on millisecond to minute timescales [18] , [19] , spontaneous emission lifetimes ( T 1 ) of 20 to 200 ps [5] , [7] , [12] , [17] , [20] and ultrafast exciton decoherence or dephasing time ( T 2 ) of up to about 500 fs till date [21] , [22] . So far, exciton dephasing has only been investigated in ensemble studies, which are likely affected by surfactants, inter-tube and tube–substrate coupling effects. The question arises to what extent these experiments probe the true intrinsic properties of the exciton dynamics and how one could reach deeper into the intrinsic regime. In particular, theorists predicted about a decade ago T 1 times of excitons of about 10 ns (refs. 23 , 24 ) while measurements have lifetimes varying from <20 to 200 ps. Recently, Perebeinos and Avouris [25] proposed a mechanism that attributes this discrepancy to residual p -type doping opening up an efficient non-radiative recombination channel via phonon-assisted indirect exciton ionization (PAIEI). This implies that the ps-fast T 1 times are extrinsic and that intrinsic exciton properties could be expected when doping is reduced. To this end, it is appealing to study SWCNTs that are isolated from their environment by suspending them over an air gap, as previously performed by one of the authors [26] . Such elevated SWCNTs are often said to be ultra-clean, to reflect the reduced disorder in the absence of a substrate, which facilitated the observation of phenomena such as Wigner crystallization [27] , spin-orbit coupling [28] and the Mott insulating state [26] . Recent optical studies of air-bridged SWCNTs have shown that this approach can also eliminate blinking and SD on the millisecond to minute timescales [29] , and an indirect estimate of the T 2 dephasing times from the spectral linewidth was reported [30] . However, as the linewidth can be in principle affected by SD, it is not a reliable measure for exciton dephasing and only a lower temporal bound. Direct measurements of exciton dephasing in the time domain have not yet been carried out for individual SWCNTs. Here we report time-resolved PL measurements over 14 orders of magnitude for individual ultra-clean SWCNTs bridging an air gap over pillar posts. Our cryogenic single nanotube measurements demonstrate a new regime of intrinsic localized exciton photophysics with narrow spectral linewidth down to 200 μeV and prolonged spontaneous emission times up to 18 ns, approaching into the intrinsic regime. In addition, we establish for the first time the exciton dephasing times for individual SWCNTs in the time domain and found fourfold prolonged values up to T 2 =2.1 ps when compared with ensemble measurements. Furthermore, our experiments demonstrate that the spectral linewidth is not a reliable measure for the exciton dephasing time in environment-affected SWCNTs of prior studies. Exciton emission from ultra-clean air-bridged SWCNTs In order to investigate the exciton photophysics without distortion from a dielectric surrounding or surfactants, we have grown SWCNTs in such a way that they bridge an air gap between pillar posts. 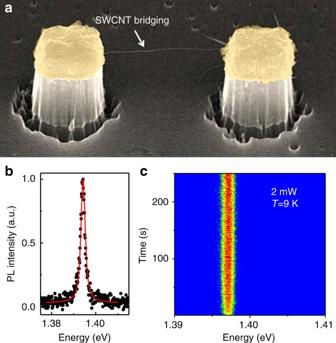Figure 1: Optical emission from individual air-bridged SWCNTs. (a) Scanning electron microscope image of an individual SWCNT bridging two pillar posts, which are separated 3 μm from centre to centre. The directional growth starts from the Co metal catalyst located on top of the pillars (shaded yellow). (b) PL spectrum of an individual and pristine SWCNT with (6,4) chirality suspended in air. Symmetric lineshapes are observed at 9 K and pump powers of 50 μW. Solid red line is a Lorentzian fit. (c) Spectral trajectory of the PL emission recorded with 200-ms timing resolution showing no significant SD and blinking at this timing resolution. Figure 1a shows a corresponding scanning electron micrograph image of an individual SWCNT with a length of about 2 μm. The CNT nucleation starts predominantly from a Co-layer deposited on top of the pillars acting as a catalyst. The growth direction follows the gas-flow stream until the other end is reached [15] , [31] . More details are given in the Methods section. From scanning electron microscope scans of about 1,000 pillar post pairs, we determine a success rate of 15% that an individual SWCNT is fully elevated. In some cases, the SWCNT would grow from the top diagonal down to the substrate but still being elevated along its entire length, while in most cases the location is simply empty. As a result, spatial scans in micro-PL reveal single narrow emission lines in the spectrum in case of semiconducting SWCNTs. In addition, the emission lines display pronounced intensity dependence upon rotation of the linear incident laser polarization, indicating that the optical emission stems from individual SWCNTs [18] , [19] . The spectrum in Fig. 1b demonstrates single Lorentzian lineshapes of the E 11 exciton recombination and the corresponding spectral trajectory in Fig. 1c shows that the emission is stable with no significant SD or blinking at 200-ms timing resolution. The 890-nm emission wavelength is attributed to SWCNTs with (6,4) chirality [32] . While we find SWCNTs with various chiralities along the wafer, we focus here on the (6,4) tubes to avoid any potential variations in the exciton photophysics due to differences in the tube diameter. Figure 1: Optical emission from individual air-bridged SWCNTs. ( a ) Scanning electron microscope image of an individual SWCNT bridging two pillar posts, which are separated 3 μm from centre to centre. The directional growth starts from the Co metal catalyst located on top of the pillars (shaded yellow). ( b ) PL spectrum of an individual and pristine SWCNT with (6,4) chirality suspended in air. Symmetric lineshapes are observed at 9 K and pump powers of 50 μW. Solid red line is a Lorentzian fit. ( c ) Spectral trajectory of the PL emission recorded with 200-ms timing resolution showing no significant SD and blinking at this timing resolution. Full size image Interestingly, we do not find any evidence of asymmetric exciton lineshapes ( Supplementary Fig. S1 ) with linewidth of about 3.5 meV as previously reported for surfactant-embedded SWCNTs grown by the CoMoCat technique, which were attributed to an intrinsic dephasing mechanism of excitons and acoustic phonons [33] . Such an asymmetry was also reported for air-bridged SWCNTs displaying rather large linewidth of 10 meV and attributed to the Van Hove singularities in the density of states [34] . The relatively large linewidth of 10 meV in the absence of a substrate as found in Lefebvre et al . [34] is also indicative that even air-bridged SWCNTs can be affected by the environment, possibly owing to residual unintentional doping. To shine more light on this issue, we targeted the growth of ultra-clean SWCNTs with the idea that shorter growth time should result in less residual amorphous carbon in the SWCNT vicinity. In Fig. 2 , we compare the spectral linewidth as a function of pump power for surfactant-dispersed SWCNTs of (6,4) chirality embedded in a polystyrene matrix (blue triangles), with air-bridged SWCNTs grown for 10 min (black squares) and air-bridged SWCNTs grown for only 2 min (red circles). Compared with surfactant-dispersed SWCNTs with linewidth up to 10 meV, the air-bridged SWCNTs from the 10 min growth are significantly narrower. Best values down to 220 μeV are found in the 2 min growth run. As it is well known that charge fluctuations from residual doping can give rise to SD resulting in linewidth broadening [18] , [19] , one can conclude that observation of ultra-narrow spectral emission lines in the 2 min growth is caused by ultra-clean SWCNTs. 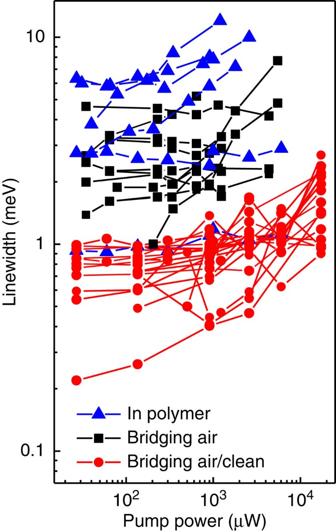Figure 2: Spectral linewidth study. Linewidth versus pump power for surfactant-dispersed and polymer-embedded SWCNTs (blue triangles), air-bridged SWCNTs grown for 10 min (black squares) and ‘cleaner’ air-bridged SWCNTs grown for only 2 min (red circles). All data are corrected for the spectrometer response function by fitting a Voigt function to the time-integrated spectrum, that is, a convolution of a single Lorentzian describing the exciton recombination and a Gaussian describing the system broadening. Data are recorded at 9 K. Figure 2: Spectral linewidth study. Linewidth versus pump power for surfactant-dispersed and polymer-embedded SWCNTs (blue triangles), air-bridged SWCNTs grown for 10 min (black squares) and ‘cleaner’ air-bridged SWCNTs grown for only 2 min (red circles). All data are corrected for the spectrometer response function by fitting a Voigt function to the time-integrated spectrum, that is, a convolution of a single Lorentzian describing the exciton recombination and a Gaussian describing the system broadening. Data are recorded at 9 K. Full size image The narrow and symmetric lineshape implies that the proposed acoustic-phonon dephasing mechanism giving rise to asymmetric and broader lineshapes is either not intrinsic, that is, substrate, dopant and/or surfactant induced, or not relevant at a comparable magnitude when SWCNTs are suspended in air. In particular, our observation of a spectral linewidth of 220 μeV implies a lower limit for the dephasing time T 2 of 6 ps, which is about an order of magnitude longer than previously assumed. In addition, one can expect that the spontaneous emission lifetime T 1 becomes significantly longer if the PAIEI non-radiative decay channel is effectively suppressed in ultra-clean SWCNTs. SD via photon correlation spectroscopy To further investigate the photophysics of excitons in these air-bridged SWCNTs and demonstrate prolonged T 1 and T 2 times as the signature of the intrinsic regime, we carried out time-resolved measurements over 14 orders of magnitude from minutes down to the sub-ps regime. The emission energy and intensity of the exciton recombination of an individual quantum emitter is well known to strongly fluctuate with time due to SD and blinking, which can give rise to significant linewidth broadening and low quantum efficiency. These detrimental quantum fluctuations are, however, to a large part not intrinsic and can be strongly suppressed, either by embedding SWCNTs into a polystyrene matrix as we have shown recently [18] , [19] or by dispersing the SWCNT in air [29] . Our data from the air-bridged SWCNTs shown in Fig. 1c confirm these earlier findings, that is, there are no pronounced effects of SD or blinking even for the 10-min growth samples when streaming photons for 5 min at a timing resolution of 100 ms. However, such studies of SD and blinking based on direct streaming of the photon flux with CCD cameras or single photon avalanche photodiodes (APDs) are limited to timescales of ms or μs at best. This raises the question if the residual linewidth of air-suspended SWCNTs is affected by SD on faster timescales, which are not resolved in these experiments. In order to investigate such contributions of SD down to the ns timescale, we describe in the following an experiment based on photon correlation spectroscopy [18] , [35] applied here for the first time to air-suspended SWCNTs. 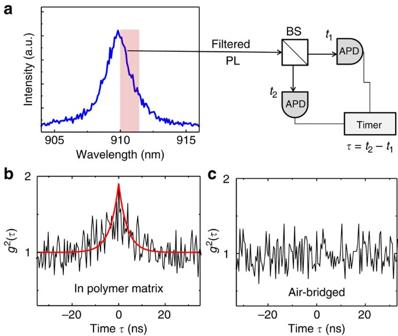Figure 3: SD studies using photon correlations measurements. (a) Plot of PL emission spectrum of an individual polymer-embedded SWCNT (blue line). Spectrally filtered light (pink-shaded bandpass) is directed to a photon coincidence setup (BS, beam splitter; APD, avalanche photodiode). (b,c) Corresponding plots of the second-order photon correlation function under continuous wave excitation. Trace (b) was recorded with a 10 nm filter centred over the right half of the emission spectrum shown in (a) for a polystyrene-embedded SWCNT. The red line is a fit to a rate equation described in the text and detailed in Walden-Newmanet al.18The photon bunching signature with a decay time of 3.7±0.4 ns is a measure for the SD time. Bunching is absent in trace (c) even with 1 nm narrow filtering for a pristine SWCNT bridging an air gap. Pump power is 200 μW for (a) and 1.8 mW for (b). All measurements were taken at 9 K. Figure 3a illustrates the measurement principle: we assume that the measured PL spectrum (blue) is composed of intrinsically much narrower spectral lines that rapidly fluctuate around a centre wavelength due to SD. By sending light from a specific subregion of the PL spectrum selected by a bandpass filter (pink-shaded area) towards the single photon correlation setup, one creates a conditional detection probability that a second photon will be detected from the same spectral region at a later time. This detection probability eventually decreases with time if the exciton recombination energy shifts out of the spectral detection window due to SD, that is, the optical Stark shift generated by fluctuating charges. As a result, the signature of SD in the second-order photon correlation function g 2 ( τ ) is a bunching signal centred at zero delay time decaying with the characteristic SD time. Figure 3: SD studies using photon correlations measurements. ( a ) Plot of PL emission spectrum of an individual polymer-embedded SWCNT (blue line). Spectrally filtered light (pink-shaded bandpass) is directed to a photon coincidence setup (BS, beam splitter; APD, avalanche photodiode). ( b , c ) Corresponding plots of the second-order photon correlation function under continuous wave excitation. Trace ( b ) was recorded with a 10 nm filter centred over the right half of the emission spectrum shown in ( a ) for a polystyrene-embedded SWCNT. The red line is a fit to a rate equation described in the text and detailed in Walden-Newman et al . [18] The photon bunching signature with a decay time of 3.7±0.4 ns is a measure for the SD time. Bunching is absent in trace ( c ) even with 1 nm narrow filtering for a pristine SWCNT bridging an air gap. Pump power is 200 μW for ( a ) and 1.8 mW for ( b ). All measurements were taken at 9 K. Full size image For comparison, we first illustrate in Fig. 3b a SWCNT that has been dispersed in a surfactant and embedded in a polymer matrix (see Methods). This SWCNT displays pronounced bunching when filtered with a 10 nm bandpass centred over the right half of the emission spectrum. The bunching disappears when filtered with a 40-nm-wide filter covering the entire PL spectrum as expected, as in this case no conditional probability is created at the detector. The SD decay time can be quantified using the relation , where γ L,R is the crossover rate for shifting in and out of the filter range, which determines the peak height, and γ d is the SD rate, which determines the SD time τ d =1/ γ d . From the solid red curve fit of g 2 ( τ ) in Fig. 3b , we find τ d =3.7±0.4 ns. These SD times vary as a function of pump power, as well as dielectric environment, and are most pronounced in uncapped SWCNTs touching a SiO 2 substrate, as further detailed in Walden-Newman et al . 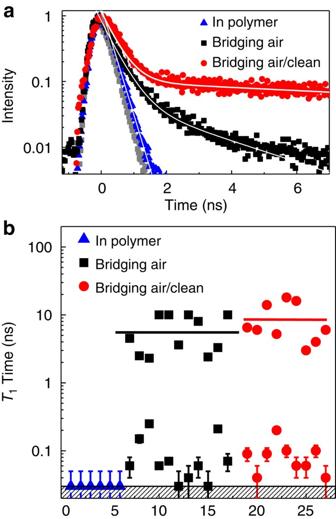Figure 4: Spontaneous emission time recorded by time-correlated single photon counting. (a) PL intensity as a function of delay time after pulsed excitation at 780 nm into a phonon sideband. The grey squares are the system response recorded for backreflected laser light and fit by a monoexponential function with decay time of 210 ps. All polymer-embedded samples are nearly resolution limited (blue triangles) and fit by a monoexponential function (white line) with a deconvolved decay time of 30±20 ps. The error bars (±20 ps) correspond to the uncertainty in determining the lifetime in the monoexponential fit. Air-bridged SWCNTs from 10 min growth (black squares) and 2 min growth (red circles) are fit by a biexponential function (white lines) with a faster component of 30–200 ps and a slower component of several ns. (b) Overview of fittedT1times versus number of investigated SWCNT. Horizontal lines indicate average values of the slow component. Data are recorded at 9 K. [18] Figure 4: Spontaneous emission time recorded by time-correlated single photon counting. ( a ) PL intensity as a function of delay time after pulsed excitation at 780 nm into a phonon sideband. The grey squares are the system response recorded for backreflected laser light and fit by a monoexponential function with decay time of 210 ps. All polymer-embedded samples are nearly resolution limited (blue triangles) and fit by a monoexponential function (white line) with a deconvolved decay time of 30±20 ps. The error bars (±20 ps) correspond to the uncertainty in determining the lifetime in the monoexponential fit. Air-bridged SWCNTs from 10 min growth (black squares) and 2 min growth (red circles) are fit by a biexponential function (white lines) with a faster component of 30–200 ps and a slower component of several ns. ( b ) Overview of fitted T 1 times versus number of investigated SWCNT. Horizontal lines indicate average values of the slow component. Data are recorded at 9 K. Full size image In contrast, Fig. 3c demonstrates that such a bunching signature is completely absent in air-bridged SWCNTs from the 10 min growth. The experiment was carried out at a pump power of 1.8 mW were the particular SWCNT displays a spectral linewidth of 2.2 meV (1.4 nm), which was filtered with a 1-nm bandpass filter positioned over the right half of the emission spectrum. By recording the transmitted spectrum in each arm before APDs, we confirmed that a conditional probability is created (see Supplementary Fig. S2 ). We tested more than 20 air-bridged SWCNTs and never found bunching while every surfactant-dispersed SWCNT did reliably produce a bunching signature. As a result, the photon correlation experiments reveal that there are no contributions of SD in air-bridged SWCNTs down to the system resolution limit of about 200 ps. One reason why the correlation trace for the air-bridged tubes does not show bunching from residual SD could be that it is masked by photon antibunching from localized quantum-dot-like excitons. Measurements with a 10-nm-broad filter before detectors can exclude this as an explanation ( Supplementary Fig. S3 ). Therefore, our measurements show that either there is no SD or, which is more likely in light of our findings in Fig. 5e , that residual SD contributes to the linewidth, but is much faster than what can be resolved with the correlation technique. 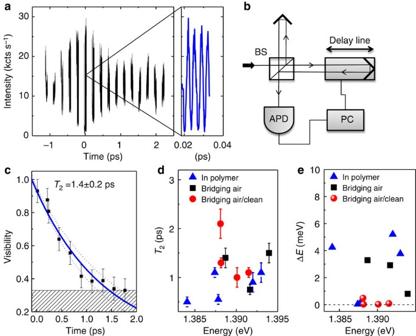Figure 5: Exciton dephasing time measurements of individual SWCNTs using a Michelson interferometer. (a) Intensity as a function of delay time between the two beams in the interferometer. The right panel magnifies the pronounced fringe contrast near zero delay time. (b) Schematic of Michelson interferometer using retro mirrors on a delay line. BS, beam splitter; APD, avalanche photodiode; PC, computer control. (c) Fringe visibility as a function of delay time recorded at 9 K for a pristine SWCNT bridging an air gap (black dots). The blue solid line is a monoexponential decay fit. The error bars highlight the uncertainty in the analysis of the fringe contrast. The dashed lines indicate the resulting spread when fitting the fringe decay monoexponential, which is ±0.2 ps in this case. (d) Dephasing times for individual SWCNTs in polymer (blue triangles), bridging air for 10 min growth (black squares) and bridging air for 2 min growth (red circles). Error bars correspond to the spread when fitting the fringe decay monoexponential. (e) Energy difference (ΔE) between SWCNTs linewidth determined from PL spectra and corresponding linewidth of the measuredT2data from panel (d). Data are recorded at 9 K and pump power of about 900 μW. Figure 5: Exciton dephasing time measurements of individual SWCNTs using a Michelson interferometer. ( a ) Intensity as a function of delay time between the two beams in the interferometer. The right panel magnifies the pronounced fringe contrast near zero delay time. ( b ) Schematic of Michelson interferometer using retro mirrors on a delay line. BS, beam splitter; APD, avalanche photodiode; PC, computer control. ( c ) Fringe visibility as a function of delay time recorded at 9 K for a pristine SWCNT bridging an air gap (black dots). The blue solid line is a monoexponential decay fit. The error bars highlight the uncertainty in the analysis of the fringe contrast. The dashed lines indicate the resulting spread when fitting the fringe decay monoexponential, which is ±0.2 ps in this case. ( d ) Dephasing times for individual SWCNTs in polymer (blue triangles), bridging air for 10 min growth (black squares) and bridging air for 2 min growth (red circles). Error bars correspond to the spread when fitting the fringe decay monoexponential. ( e ) Energy difference (Δ E ) between SWCNTs linewidth determined from PL spectra and corresponding linewidth of the measured T 2 data from panel ( d ). Data are recorded at 9 K and pump power of about 900 μW. Full size image Prolonged spontaneous emission lifetimes With this clear advantage of air-bridged SWCNTs compared with surfactant-dispersed SWCNTs, one can now examine the intrinsic properties of the exciton photophysics. In particular, we expect that the spontaneous emission time T 1 approaches the intrinsic limit of several ns, which was theoretically predicted by Perebeinos and Avouris [25] for the case of moderate exciton localization and when PAIEI can be neglected. The PAIEI mechanism is caused by unintentional doping pinning the Fermi level in the valence band, which opens up a very effective non-radiative decay channel via phonon-assisted intraband electron–hole pair generation. In this sense, the absence of SD down to sub-ns timescales in Fig. 3c , as well as the narrow spectral linewidth in Fig. 2 , is very promising, implying a lower residual dopant concentration and thus suppressed PAIEI as compared with surfactant-dispersed SWCNTs. The dynamics of the exciton recombination was recorded by time-correlated single photon counting as shown in Fig. 4 . For our comparison group of surfactant-dispersed SWCNTs, we find in all cases nearly resolution-limited T 1 times, as shown in Fig. 4a (blue triangles). After deconvolution of the system response function (210 ps), an upper bound for the T 1 times of about 30±20 ps is estimated. In stark contrast, all investigated air-bridged SWCNTs display a pronounced biexponential decay behaviour ( Fig. 4a ), with a moderately long T 1 time of 30–200 ps and a second ultra-long decay time of up to 10 ns for the 10 min growth, and up to 18 ns for the 2 min growth. Statistical results recorded from 20 individual air-bridged SWCNTs are shown in Fig. 4b . Average values of the 10 min growth are found to be T 1 =5.7 ns and for the 2 min growth T 1 =9 ns, as indicated by the horizontal lines. As a result for the three groups of SWCNTs, narrower linewidth as shown in Fig. 2 correlates with longer T 1 times as shown in Fig. 4 . This strongly indicates that the effective removal of unintentional doping gradually removes the PAIEI decay channel, giving rise to the observed ns decay component. The pronounced variation of T 1 times in the air-bridged SWCNTs from 4 to 18 ns and the contribution of a 30 to 200-ps-fast component are attributed to the varying degree of exciton localization and any residual unintentional doping. From transport measurements of comparable SWCNTs grown in the same chemical vapour deposition furnace, it is known that the electron mean free path varies between 400 nm and 10 μm, recorded at 10 K where one can neglect contributions from acoustic phonons to transport [36] . These variations in the electron mean free path have been attributed to the static disorder caused by residual impurities and they correlate with the number of defects determined from scanning gate microscopy [36] . Therefore, if a particular section along the tube is less affected by residual doping, the PAIEI mechanism responsible for the 30 to 200-ps-fast non-radiative decay is effectively suppressed, while excitons in other sections of the SWCNT can still recombine fast. In the clean sections and absence of PAIEI, the T 1 time is only adversely affected by intrinsic multiphonon decay, which strongly varies in presence of exciton localization. Calculations of T 1 times for SWCNT with diameter of 1 nm predict T 1 values of 100 ns in the absence of exciton localization, which speeds up to about 0.5 ns for strong exciton localization along the tube [25] . Therefore, our measured T 1 values of 4 to 18 ns reveal the onset of a remarkable new regime of intrinsic localized exciton recombination approaching spontaneous emission times predicted about a decade ago by theorists [23] , [24] . Prolonged exciton dephasing Finally, we present exciton dephasing measurements for the first time for individual SWCNTs in the time domain by recording the first-order autocorrelation function g 1 ( τ ) with a Michelson interferometer. Figure 5a shows the interferogram of light from the E 11 exciton recombination. The right panel illustrates the high fringe visibility with values up to 97% achieved by a delay line with retro mirrors ( Fig. 5b ) and a stepping resolution of 50 nm. The fringe visibility V ( τ ) was estimated using the relation V ( τ )=( I max ( τ )− I min ( τ ))/( I max ( τ )+ I min ( τ )), where I max ( τ ) and I min ( τ ) are the fringe maxima and minima determined from fits to the fringe pattern at various delay times. Figure 5c shows V ( τ ) as a function of delay time, which fits monoexponentially with decay time T 2 =1.4±0.2 ps. At a fringe visibility at or below 35%, the data become too noisy to be reliable, constituting the detection limit, as indicated by the black shading. Dephasing times determined in this way are plotted in Fig. 5d for all three cases. While surfactant dispersed, polymer-embedded SWCNTs show on average the fastest dephasing with 830 fs, air-bridged SWCNTs from the 10 min growth display an average T 2 =1.22 ps, while the cleaner 2 min growth yields an average of T 2 =1.38 ps with a longest value of T 2 =2.1 ps, which corresponds to a fourfold prolonged exciton dephasing time when compared with ensemble measurements [21] , [22] . Our linewidth measurements down to 220 μeV at lowest pump power imply furthermore a lower limit of 6 ps for the T 2 time of the air-bridged SWCNTs from the 2 min growth. The interferometric measurements at the level of individual SWCNT require, however, larger pump powers resulting in broader linewidth ( Fig. 2 ), limiting the experimental accessible range for T 2 measurements to the high pump powers. It is interesting to compare exciton dephasing times estimated by the direct time-domain approach with the indirect frequency-domain measurements, that is, the spectral linewidth of the PL emission. If there is no other physical mechanism affecting the spectral linewidth, such as SD, then both values from time- and frequency-domain experiment should match and follow the well-known relation . For this purpose Fig. 5e plots the difference in energy between the measured spectral PL linewidth and the spectral linewidth, which can be estimated with the above relation from the measured T 2 values from Fig. 5d . In estimating the linewidth, we corrected for possible broadening from the T 1 process, which is, however, a rather small correction, such that is dominated by the dephasing time alone ( Supplementary Fig. S4 ). The deviations for polymer-embedded SWCNTs up to 6 meV and air-bridged SWCNTs from the 10 min growth up to 3.7 meV in Fig. 5e are striking and imply that the exciton dephasing time in SWCNTs cannot be accurately determined from a time-integrated linewidth study alone, as was previously suggested [30] . In contrast, our ultra-clean samples from the 2 min growth show little to no extra broadening in Fig. 5e (red dots), thus following the standard relation . This is another clear indication that emission from the samples of the 2 min growth approaches the intrinsic regime. We furthermore note that the measured lifetimes of T 1 =4–18 ns are indicative of localized exciton emission as calculations of T 1 times for SWCNT with diameter of 1 nm predict T 1 values of 100 ns in the complete absence of exciton localization, which speeds up to about 0.5 ns for strong exciton localization along the tube [25] . One would thus expect that the localization can result in quantum-dot-like states along the nanotube, which should give rise to nonclassical light emission in form of photon antibunching. While we do find pronounced signatures of photon antibunching under pulsed excitation in several polymer-embedded SWCNTs, as well as air-bridged SWCNTs (see Supplementary Figs S5 and S6 ), we find also many air-bridged SWCNTs that do not display photon antibunching despite their narrow linewidth and prolonged T 1 and T 2 times. As SWCNTs can possess several localization sites along the tube length, and as the optical excitation spatially averages over them, the photon antibunching signatures can vanish in the limit of several quantum emitters. On the other hand, all air-bridged SWCNTs display contributions of prolonged T 1 times, which have been predicted about a decade ago by theorists [23] , [24] , and are the hallmark of the intrinsic exciton recombination. Finally, we discuss the underlying dephasing mechanism in light of our new findings. It is well known that optical phonons dominate the exciton dephasing above a lattice temperatures of 180 K (ref. 22 ), while at our cryogenic measurement temperatures of 9 K exciton dephasing is dominated by one-phonon acoustic scattering with a linear bath temperature dependence [21] , [22] , [30] , [33] . Other processes such as collision-induced broadening from elastic exciton–exciton scattering and exciton–exciton annihilation provide an additional contribution to the exciton dephasing, which is, however, rather small at intermediate pump powers were our experiments are carried out, while values reach up to 100 μeV in the high pump power saturation regime [37] . A recent theory also predicts suppression of exciton–electron scattering in doped SWCNTs for the optically active singlet exciton at low temperatures with contributions to dephasing of 100 μeV or less at 50 K and high doping (0.3 electrons per nm), which vanishes at low doping levels [38] . The merit of our finding is that the magnitude of the exciton acoustic-phonon scattering is sizably smaller than concluded in prior reported efforts. This is evident from both the remarkably narrow linewidth ( Fig. 2 ) and the prolonged dephasing times ( Fig. 5 ), which we observed for the first time in our experiments. As an example of prior efforts, Galland et al . [33] finds asymmetric spectral lineshapes with 3.5 meV linewidth ( T 2 about 400 fs) and applies the independent Boson model to fit the lineshape based on the magnitude of the exciton–phonon matrix elements g j ( q ), which is a product of the exciton form factor F ( q ) describing coupling in momentum space and the deformation potential coupling G s ( q ) of the stretching mode. Agreement between theory and experiment has been found using a deformation potential value for the stretching mode of D s =12–14 eV and an exciton wavefunction envelope of about 10 nm. It is, however, also clear that these parameters can depend strongly on the nanotube environment. On one hand, in F ( q )=exp(− q 2 σ 2 /4), the exciton confinement length σ depends on the underlying degree of exciton localization, which can vary from tube to tube and in different environments [39] . On the other hand, G s ( q ) depends linearly on D s and inversely on the square root of the SWCNT length. The magnitude of the deformation potential coupling is likely smaller in air-bridged SWCNT, as for a substrate-supported SWCNT the effective deformation potential can be additionally affected by substrate phonons. This is, for example, the case in graphene on SiO 2 showing strongly reduced carrier mobility owing to scattering with interface phonons, while air-suspended graphene displays an order of magnitude larger mobility. Besides acoustic phonons, disorder and/or structural defects contribute additionally to the exciton dephasing. Ab initio calculations of (6,4) SWCNTs predict that Stone–Wales or 7557-type defects can introduce a broad range of disorder modes resulting in fast exciton dephasing down to 10 fs at room temperature [40] . It is thus likely that amorphous carbon or graphitic residue decorating the SWCNT can also contribute to the exciton dephasing, in particular as the weak Coulomb screening allows the exciton wavefunction to penetrate into the tube vicinity. Our remarkably narrow spectral linewidth and the prolonged dephasing time for the air-bridged SWCNTs from the 2 min growth suggest that they have significantly lower disorder and defects than prior efforts. As a result, our data show that the intrinsic exciton acoustic-phonon coupling in ultra-clean air-bridged SWCNTs is significantly weaker than previously believed, while the presence of disorder from residual amorphous carbon or defects can give rise to SD and faster exciton dephasing times, even in some of the air-bridged SWCNTs. In summary, we carried out time-resolved PL measurements over 14 orders of magnitude for individual SWCNTs bridging an air gap over pillar posts. Our measurements demonstrate a new regime of intrinsic localized exciton photophysics in ultra-clean SWCNTs displaying prolonged spontaneous emission times up to T 1 =18 ns, which have been predicted by theorists about a decade ago. Longer lifetimes are attributed to an effective suppression of phonon-assisted indirect exciton dissociation, the PAIEI mechanism, which can be caused by unintentional doping. This is in agreement with photon correlation experiments demonstrating that surfactant-dispersed SWCNTs display SD while air-bridged SWCNTs are free of SD down to the detection limit, implying reduced background doping. Furthermore, we measured for the first time the exciton dephasing times for individual SWCNTs in the time domain and found fourfold prolonged values up to T 2 =2.1 ps compared with ensemble measurements. Our experiments demonstrate that the spectral linewidth is not a reliable measure for the exciton dephasing time in prior SWCNTs, unless ultra-clean SWCNTs reach deeply into the intrinsic regime. The ultra-narrow linewidth and prolonged dephasing times suggest that the matrix element for exciton acoustic-phonon coupling has been largely overestimated in previous work. While a longer dephasing is of importance for applications in quantum optics, the prolonged exciton dynamics is promising towards efficient optoelectronic and quantum photonic devices based on ultra-clean SWCNTs. Sample preparation In order to create elevated SWCNTs bridging an air gap, a 1-nm-thin layer of Co was deposited by electron-beam evaporation onto a Si/SiO 2 wafer. Pillar pairs of 3 μm spacing and lateral walls of 5 μm spacing were defined lithographically and transferred by reactive-ion etching into the Si/SiO 2 /Co substrate for about 2.5 μm. SWCNTs were grown by ambient chemical vapour deposition method using a modified fast-heating process with ethanol as feedstock [41] , [42] . Growth was carried out at a temperature of 900 °C in an Ar/H 2 gas mixture at typical EtOH flow rates of 80 s.c.c.m. The pillar pairs were spaced out 30 μm in order to avoid any unwanted emission from neighbouring SWCNTs in the optical measurements. The growth time was varied between 2–10 min. For comparison studies, we also used commercial SWCNTs grown by the CoMoCat technique, which were embedded in polystyrene on top of a gold mirror to enhance outcoupling. These samples were fabricated using an ebeam evaporator to coat a 100 nm layer of Au on top of a standard p++ type Si wafer with a 90 nm SiO 2 layer. This was followed by a 160 nm layer of spin-coated polystyrene. Commercial CoMoCat SWCNTs were prepared with bath sonication for 1 h in a vial containing 0.4 wt % SDS solution. The product was poured through a 5 μm filter to form a concentration of 0.2 mg ml −1 , and deposited directly onto the first layer of polymer, and then covered with a second 160 nm layer of polymer. Finally, the samples were baked at 95 °C for several hours before cryogenic measurements to remove moisture acting as charge trap states [43] . This approach effectively removes SD and blinking as we recently demonstrated [18] , [19] . Micro-PL setup Measurements of micro-PL (μ-PL) were taken inside a liquid helium cryostat with a 9 K base temperature. Samples were excited with a laser diode operating at 780 nm in continuous wave or pulsed mode (80 MHz repetition rate and 100-ps pulse length). A laser spot size of about 1.5 μm was achieved using a microscope objective with numerical aperture of 0.55. The relative position between sample and laser spot was adjusted with a piezo-electric xyz -actuator mounted directly onto the cold finger of the cryostat. Spectral emission from the sample was dispersed using a 0.75 m focal length spectrometer and imaged by a liquid nitrogen cooled CCD camera. Laser stray light was rejected combining a 780 nm notch filter and 800 nm high-pass filter. To enhance the exciton emission, the laser polarization was rotated with a half-wave plate with respect to the axis of the SWCNTs. Measurements of spectral trajectory over time were obtained by continuously recording the spectra every 200 ms with a silicon CCD camera. Photon correlation measurements The second-order photon correlation function g 2 ( τ ) was recorded by sending the PL emission through narrow bandpass filters and onto a Hanbury–Brown and Twiss setup consisting of a fibre-coupled 50/50 beam splitter connected to two single photon counting avalanche photodiodes (silicon APD). A linear polarizer was used in the collection path for photon antibunching measurements and narrow bandpass filters for the SD measurements. Coincidence counts were time stamped and analysed with a high-resolution timing module. To determine spontaneous emission lifetimes ( T 1 ), the 50/50 beam splitter was removed and the first-order photon correlation function g 1 ( τ ) was recorded by sending light from the sample to the first detector (start) and an electronic trigger from the 780-nm laser diode to the stop channel on the timing module. The system response function was measured sending scattered laser light from the sample surface to the start APD. How to cite this article: Sarpkaya, I. et al . Prolonged spontaneous emission and dephasing of localized excitons in air-bridged carbon nanotubes. Nat. Commun. 4:2152 doi: 10.1038/ncomms3152 (2013).